Germination and infectivity of microconidia in the rice blast fungusMagnaporthe oryzae The rice blast fungus Magnaporthe oryzae is a model for studying fungal–plant interactions. Although it produces two types of spores (microconidia and macroconidia), previous infection studies have exclusively dealt with macroconidia. Germination of microconidia has not been reported, and their role in plant infection is not defined. Here we show that approximately 10% of microconidia germinate on plant surfaces, and that colonies derived from germinated microconidia are normal in growth and pathogenesis. In infection assays with rice and barley seedlings, microconidia fail to infect intact plants, but they can colonize and develop necrotic lesions on wounded leaves and stems. Microconidia also cause disease symptoms on inoculated spikelets in infection assays with barley and Brachypodium heads. Furthermore, microconidia are detected inside rice plants that developed blast lesions under laboratory or field conditions. Therefore, microconidia can germinate and are infectious, and may be an important factor in the rice blast cycle. Rice blast caused by the ascomycete Magnaporthe oryzae is one of the most destructive diseases of rice worldwide and one of the top 10 fungal diseases that threaten global food security [1] . In the past two decades, it has been developed as a model system to study fungal–plant interactions [2] , [3] . In addition, species closely related to M. oryzae infect different grass species and cause other important plant diseases, including wheat take-all and grey leaf spot of turfgrass. In recent years, wheat blast caused by an emerging M. oryzae isolate has spread through South America and now poses a serious threat to wheat production [4] , [5] . Many plant pathogenic fungi are ascomycetes that produce more than one type of asexual spores. The rice blast fungus produces both microconidia and macroconidia [6] , [7] . However, to date, all the infection studies exclusively dealt with macroconidia. In general, infection of rice plants by M. oryzae is considered to be initiated by the attachment of macroconidia (often simply referred to as conidia) to plant surfaces. Germ tubes emerging from macroconidia develop melanized appressoria to physically penetrate plant cuticle and cell wall [2] , [8] . After penetration, invasive hyphae grow biotrophically in host cells at early infection stages [9] , [10] . In late infection stages, infectious growth of the pathogen results in plant cell death and lesion development [8] , [11] . Under favourable conditions, conidia are produced on lesions and dispersed by wind or rain splash to re-initiate the infection cycle. In the past two decades, various genetic mechanisms regulating different infection processes, including conidiation, appressorium formation and invasive growth, have been characterized in M. oryzae [2] , [8] , [9] , [12] . M. oryzae can infect all parts of rice plant but neck blast is the most destructive form of rice blast. However, neck blast of rice often reaches epidemic levels without severe leaf infection in the field, suggesting that macroconidia may be not the only inoculum in nature. Furthermore, it is not clear what is and where the inoculum for the wheat blast disease comes from. Wheat blast is a devastating disease caused by M. oryzae strains that infect flowering heads and cause head blast symptoms. Foliar symptoms were not detectable in fields destroyed by wheat blast, which is puzzling but occurred in different wheat growing regions in South America [4] , [5] . Under culture conditions, M. oryzae also produces unicellular, crescent microconidia on phialides [6] , [7] , which is different from the formation of three-celled macroconidia on conidiophores. Light has no effect on the production of microconidia that are hyaline and contain a single nucleus [6] , [7] . However, microconidia have not been observed on diseased plants and are hypothesized to function as spermatia during sexual reproduction. To date, germination of microconidia has not been reported in M. oryzae . The function of its microconidia in plant infection and the blast disease cycle, if any, has not been established. Here, we show that 5–10% of microconidia can germinate on artificial and plant surfaces. Germinated microconidia can produce normal sub-cultures and infect rice or barley leaves through wounds. In infection assays with flowering barley and Brachypodium heads, microconidia are able to infect unwounded spikelets and cause disease symptoms. Furthermore, we detect microconidia produced in diseased rice plants and identify two genes that are specifically expressed in microconidia. Our results show that microconidia are infectious and they are produced in planta . Due to their smaller size, microconidia may allow M. oryzae to spread readily through the vascular system, which could be an important but neglected factor in the disease cycle and outbreaks of rice blast and other important diseases caused by Magnaporthe species. Production of abundant microconidia in liquid cultures To conduct germination and infection assays with microconidia, we first developed an efficient method to produce large amounts of microconidia in liquid cultures. Earlier publications examined microconidium production on culture plates [6] , [7] , but separating microconidia from hyphal fragments and macroconidia is problematic. 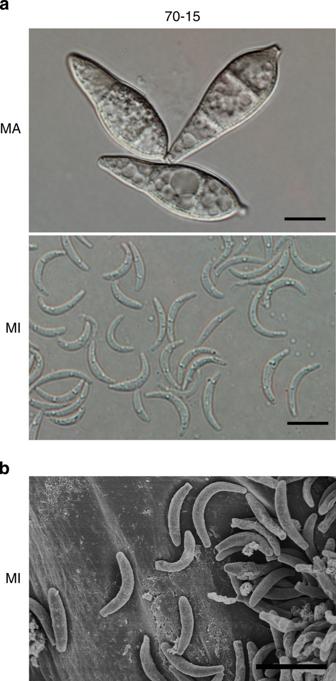Figure 1: Microconidia of the wild-type strain 70-15. (a) Microconidia (MI) and macroconidia (MA) of strain 70-15 were examined by DIC (differential interference contrast) microscopy. (b) Microconidia of strain 70-15 were examined by SEM microscopy. Scale bar, 5 μm. Because M. oryzae does not produce macroconidia in submerged cultures, we tested different liquid media and temperatures for microconidium production, and found that freshly prepared potato dextrose broth (PDB) supported the production of abundant microconidia at 20 °C ( Supplementary Table 1 ). On average, approximately 5 × 10 6 microconidia per ml were produced in 7-day-old cultures of the wild-type strain 70-15 (which was previously used for genome sequencing [13] ). The other wild-type strains P131 and Y34 (ref. 14 ) produced similar amount of microconidia under the same conditions. Microscopic examination showed that microconidia harvested from the liquid PDB cultures by filtration through Miracloth and Whatman filter paper were not contaminated with macroconidia or hyphal fragments ( Fig. 1 ). Figure 1: Microconidia of the wild-type strain 70-15. ( a ) Microconidia (MI) and macroconidia (MA) of strain 70-15 were examined by DIC (differential interference contrast) microscopy. ( b ) Microconidia of strain 70-15 were examined by SEM microscopy. Scale bar, 5 μm. Full size image The Pmk1 pathway is involved in microconidium production Because the genetic mechanism regulating the production of microconidia in filamentous ascomycetes is not clear, we examined a number of mutants that are blocked in the cyclic AMP (cAMP) and mitogen-activated protein kinase signal transduction pathways [11] , [12] for microconidium formation. The pmk1 and mst12 mutants produced over 100-fold fewer microconidia than strain 70-15. Mst12 is a transcription factor functioning downstream from the Pmk1 mitogen-activated protein kinase cascade that regulates appressorium formation [12] . The Momcm1 mutant is blocked in microconidium production on oatmeal agar cultures [15] . MoMcm1 is one of the two MADS box transcription factors that is related to appressorium formation in M. oryzae . In this study, we found that the Momcm1 mutant also failed to produce microconidia in liquid PDB cultures. Germination of microconidia is independent of nutrients After testing with different media and culture conditions, we found that microconidia failed to germinate on complete medium (CM). However, microconidium swelling and germination were observed after incubation on 1% water agar at 25 °C for 24 h. By 72 h, approximately 4.9% of microconidia produced germ tubes ( Fig. 2a ; Supplementary Movie 1 ). Although swelling of microconidia was often observed before germination, some microconidia germinated without swelling and some swollen microconidia failed to produce germ tubes. To determine why only a small percentage of microconidia germinated, microconidia were stained with 4′,6-diamidino-2-phenylindole for nuclei and Mitotracker Red for mitochondria, two fungal organelles essential for growth. As reported in an earlier study [6] , a single nucleus occupied a major portion of the intracellular space in microconidia ( Fig. 2b ). However, only approximately 9.3±4.7% of microconidia contained mitochondria in Mitotracker Red staining assays ( Fig. 2b ). The rare presence of mitochondria in microconidia was confirmed by transmission electron microscopy (TEM) examination ( Fig. 2c ). 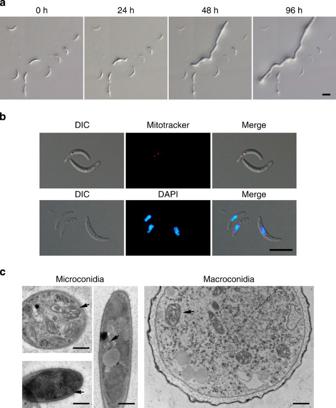Figure 2: Microconidium germination and examination for mitochondria. (a) Germination of microconidia on 1% water agar. The time lapse images of the same microconidia showing the swelling (24 h), germination (48 h) and germ tube elongation (96 h). Scale bar, 5 μm. (b) Microconidia were stained with Mitotracker Red and 4′,6-diamidino-2-phenylindole (DAPI) to observe mitochondria and nuclei, respectively. Scale bar, 5 μm. (c) Microconidia and macroconidia were examined for the presence of mitochondria (marked with arrows) by TEM. Scale bar, 500 nm. Figure 2: Microconidium germination and examination for mitochondria. ( a ) Germination of microconidia on 1% water agar. The time lapse images of the same microconidia showing the swelling (24 h), germination (48 h) and germ tube elongation (96 h). Scale bar, 5 μm. ( b ) Microconidia were stained with Mitotracker Red and 4′,6-diamidino-2-phenylindole (DAPI) to observe mitochondria and nuclei, respectively. Scale bar, 5 μm. ( c ) Microconidia and macroconidia were examined for the presence of mitochondria (marked with arrows) by TEM. Scale bar, 500 nm. Full size image Because microconidia are assumed to function as spermatia, we assayed microconidium germination in the presence of the opposite mating type. No attraction or obvious changes were observed in the germination efficiency of strain 70-15 ( MAT1-1-1 ) microconidia in the presence of germ tubes or hyphae of Guy11 ( MAT1-1-2 ) on 1% water agar ( Supplementary Fig. 1 ). The same result was obtained when we repeated this experiment on oatmeal agar, the medium used for mating assays in M. oryzae ( Supplementary Fig. 1 ). Therefore, microconidium germination and germ tube growth were not affected by the presence of a strain of the opposite mating type under the conditions tested. Viability of germinated microconidia is low Interestingly, when germinated microconidia (72 h) were transferred from water agar to CM plates, most of them (>83%) failed to develop into visible colonies ( Fig. 3a ). Those that formed colonies (approximately 17%) were normal in the production of macroconidia, appressorium formation, and plant infection, indicating that microconidia can function as propagules in M. oryzae . To determine why most germinated microconidia failed to form colonies, we assayed the viability and nuclear behaviour of microconidia germinated on 1% water agar. Close examination indicated that many germ tubes stopped further growth after the initial germination and appeared to be empty of cytoplasm or highly vacuolated by 120 h ( Fig. 3b ; Supplementary Movie 2 ). Nuclear staining also revealed that the majority (81%) of germinated microconidia had only one nucleus by 72 h ( Fig. 3c ), although approximately 14% of them eventually underwent one round of mitosis and had two nuclei in the germ tubes by 120 h ( Fig. 3c ). These results indicate that most of the germ tubes emerged from microconidia were defective in mitosis and likely underwent programmed cell death. 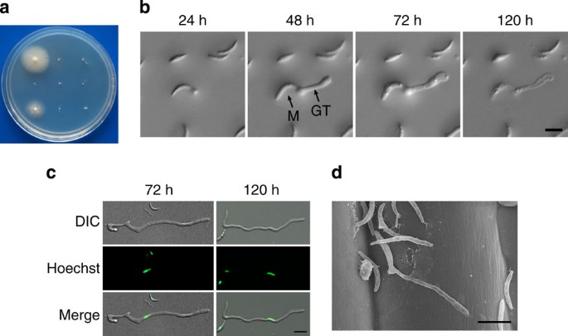Figure 3: Germ tube growth and hyphal development of microconidia. (a) Colonies formed by germinated microconidia transferred from water agar to CM. Most of them failed to develop into colonies. (b) The time lapse images of the same microconidia showing the germination and arrest of germ tube growth. Germ tubes appeared to be dead and empty of cytoplasm or highly vacuolated 120 h. M, microconidium; GT, germ tube. Scale bar, 5 μm. (c) Germinated conidia were stained with Hoechst 33258 after incubation for 72 or 120 h. Scale bar, 5 μm. (d) Microconidium germination on plant surfaces was examined by SEM at 72 h post inoculation. Scale bar, 5 μm. Figure 3: Germ tube growth and hyphal development of microconidia. ( a ) Colonies formed by germinated microconidia transferred from water agar to CM. Most of them failed to develop into colonies. ( b ) The time lapse images of the same microconidia showing the germination and arrest of germ tube growth. Germ tubes appeared to be dead and empty of cytoplasm or highly vacuolated 120 h. M, microconidium; GT, germ tube. Scale bar, 5 μm. ( c ) Germinated conidia were stained with Hoechst 33258 after incubation for 72 or 120 h. Scale bar, 5 μm. ( d ) Microconidium germination on plant surfaces was examined by SEM at 72 h post inoculation. Scale bar, 5 μm. Full size image Because autophagy has been linked to the vacuolization and collapse of macroconidium compartments after appressorium formation [16] , we isolated microconidia from the Mgatg1 mutant [17] . After germination on 1% water agar for 96 h, approximately 70% of germinated Mgatg1 microconidia were highly vacuolated and appeared to be empty and dead ( Supplementary Fig. 2 ), suggesting that autophagy is not required for cell death in germinated microconidia. Microconidia fail to form appressoria on plant surfaces We also assayed microconidium germination on plant and artificial surfaces with a transformant of 70-15 expressing green fluorescent protein (GFP) in the cytoplasm (strain GFP70). On barley leaves, germ tubes were produced by approximately 11.1±0.3% of microconidia by 72 h post inoculation when examined by scanning electron microscopy (SEM) ( Fig. 3d ) or epifluorescence microcopy ( Supplementary Fig. 3 ). This experiment was repeated at least five times. The germination rate was consistently higher on barley leaves than on 1% water agar. However, formation of appressorium-like structures was not observed in hundreds of germ tubes examined on plant surfaces. Because appressorium formation is stimulated by attachment of macroconidia to hydrophobic surfaces, we also assayed with microconidia attached to plastic coverslips for germination and appressorium formation. In repeated assays, microconidia rarely germinated on artificial surfaces but appressorium formation was never observed after incubation at 25 °C for 72 h ( Supplementary Fig. 4 ). Microconidia are infectious on wounded rice plants To determine possible functions of microconidia in plant infection, we first conducted infection assays with intact rice leaves. No lesions were formed on leaves that were sprayed or drop-inoculated with microconidia. Under the same conditions, macroconidia caused typical blast lesions ( Fig. 4a ). These results are consistent with the fact that microconidia failed to form appressoria. Lipid and glycogen staining showed that microconidia had limited carbon storage in comparison with macroconidia ( Fig. 4b ). Therefore, even if germ tubes of microconidia were able to form appressoria on plant surfaces, they lack the necessary energy reserve to generate sufficient turgor for penetration. 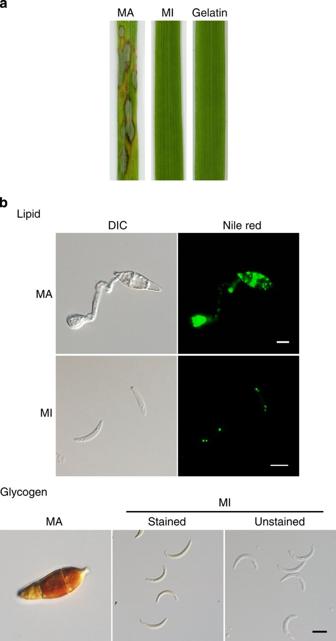Figure 4: Microconidia failed to infect intact rice leaves and had limited carbon storage. (a) Seedlings of rice cultivar Nipponbare were sprayed with macroconidia (MA) or microconidia (MI) of strain 70-15, or with 0.25% gelatin (control). Typical leaves were photographed 7 d.p.i. (b) Macroconidia (MA) and microconidia (MI) were stained for lipid bodies and glycogen. In comparison with macroconidia, microconidia had limited carbohydrate storage. Scale bar, 5 μm. Figure 4: Microconidia failed to infect intact rice leaves and had limited carbon storage. ( a ) Seedlings of rice cultivar Nipponbare were sprayed with macroconidia (MA) or microconidia (MI) of strain 70-15, or with 0.25% gelatin (control). Typical leaves were photographed 7 d.p.i. ( b ) Macroconidia (MA) and microconidia (MI) were stained for lipid bodies and glycogen. In comparison with macroconidia, microconidia had limited carbohydrate storage. Scale bar, 5 μm. Full size image Because M. oryzae mutants defective in appressorial penetration can infect through wounds, we conducted infection assays with microconidia on wounded rice plants. In rice plants injected with microconidia, no typical blast lesions were observed beyond the wound sites ( Fig. 5 ). Nevertheless, necrotic lesions were observed at 9.5% of the wound sites on leaves or leaf sheaths of rice seedlings infected by wound inoculation with microconidium suspensions ( Fig. 5a ). On rice leaves wounded by cutting or abrasion, similar results were obtained ( Fig. 5b ). When the typical necrotic lesions were excised and surface sterilized, fungal growth and conidiation were observed in most of the samples after incubation under moist conditions for 2–3 days. In plants inoculated with transformant GFP70 expressing GFP in the cytoplasm, GFP signals were observed in the M. oryzae strain recovered from the necrotic zones ( Fig. 5c ). These results indicated that although not as efficient as macroconidia, microconidia can colonize and cause disease symptoms by infection through wounds. 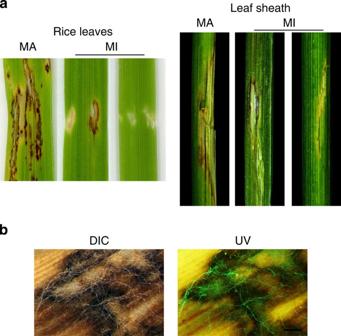Figure 5: Infection assays with wounded rice plants. (a) Rice seedlings were infected by wound inoculation with macroconidia (MA) or microconidia (MI) of strain 70-15. Disease symptoms were observed at the wounding sites on leaves (left) and sheaths (right) at 7 d.p.i. (b) Recovery ofM. oryzaefrom the necrotic zones caused by inoculation with microconidia of strain GFP70. Fungal growth and GFP signals were observed after incubation at 25 °C for 48 h. Scale bar, 500 μm. Figure 5: Infection assays with wounded rice plants. ( a ) Rice seedlings were infected by wound inoculation with macroconidia (MA) or microconidia (MI) of strain 70-15. Disease symptoms were observed at the wounding sites on leaves (left) and sheaths (right) at 7 d.p.i. ( b ) Recovery of M. oryzae from the necrotic zones caused by inoculation with microconidia of strain GFP70. Fungal growth and GFP signals were observed after incubation at 25 °C for 48 h. Scale bar, 500 μm. Full size image Infection of barley seedlings by microconidia via wounds Because barley and Brachypodium are also susceptible to M. oryzae [18] , [19] , we infected 10-day-old barley seedlings with freshly harvested microconidia. On intact barley leaves, microconidia failed to cause any lesions ( Supplementary Fig. 5 ). Under the same conditions, blast lesions were observed on leaves inoculated with macroconidia as the control. On barley leaves wounded by cutting, necrotic lesions were observed at 10.5±2.8% of the wounding sites inoculated with microconidia of GFP70 ( Fig. 6a ). When the diseased segments of barley leaves were excised and incubated in a moisture chamber for 2–3 days after surface sterilization, fungal hyphae and conidia with GFP signalling were recovered from diseased areas of barley leaves ( Fig. 6b ). These results further indicate that microconidia can infect and colonize through wounds and cause disease symptoms on wounded leaves. 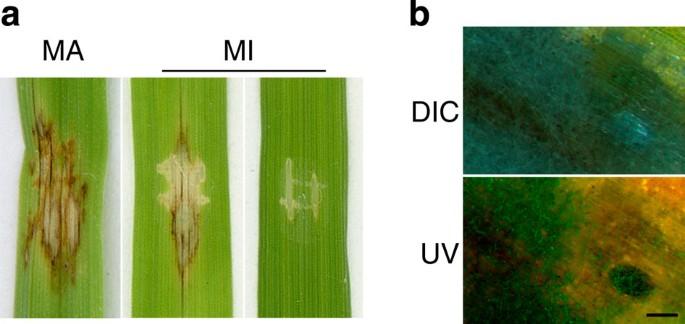Figure 6: Infection assays with wounded barley leaves. (a) Necrotic zones were observed at the wounding sites on barley leaves drop-inoculated with macroconidia (MA) or microconidia (MI) of strain GFP70 at 7 d.p.i. (b) Re-isolation ofM. oryzaefrom diseased areas caused by microconidia on barley leaves. Fungal growth and GFP signals were observed after incubation at 25 °C for 48 h. Scale bar, 500 μm. Figure 6: Infection assays with wounded barley leaves. ( a ) Necrotic zones were observed at the wounding sites on barley leaves drop-inoculated with macroconidia (MA) or microconidia (MI) of strain GFP70 at 7 d.p.i. ( b ) Re-isolation of M. oryzae from diseased areas caused by microconidia on barley leaves. Fungal growth and GFP signals were observed after incubation at 25 °C for 48 h. Scale bar, 500 μm. Full size image Microconidia are infectious on Brachypodium and barley heads We conducted infection assays with Brachypodium and barley heads because M. oryzae infects all above-ground plant parts. In Brachypodium heads drop-inoculated with microconidia, approximately 16% of the inoculated kernels became necrotic within 7–14 days post infection (d.p.i.) ( Fig. 7a ) in independent infection assays. Under the same conditions, the majority of the kernels inoculated with macroconidia developed disease symptoms ( Fig. 7a ). Discolouration of the rachis also was observed in some of the inoculated Brachypodium heads. On Brachypodium heads inoculated with GFP70, fungal hyphae and conidia with GFP signals could be isolated from diseased tissues after surface sterilization and incubation in a moisture chamber. These results indicate that microconidia, although less efficient at plant infection than macroconidia, can infect flowering Brachypodium heads by drop inoculation. 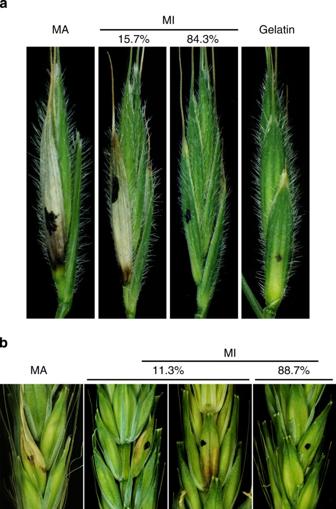Figure 7: Infection assays with Brachypodium and barley heads. Brachypodium (a) and barley (b) heads were drop-inoculated with microconidia (MI) or macroconidia (MA) of strain 70-15. Disease symptoms were examined 14 d.p.i. Inoculation with 0.25% gelatin was used as the negative control. Dots mark the inoculated kernels. On average, 15.7% of Brachypodium and 11.3% barley kernels inoculated with microconidia developed symptoms. Figure 7: Infection assays with Brachypodium and barley heads. Brachypodium ( a ) and barley ( b ) heads were drop-inoculated with microconidia (MI) or macroconidia (MA) of strain 70-15. Disease symptoms were examined 14 d.p.i. Inoculation with 0.25% gelatin was used as the negative control. Dots mark the inoculated kernels. On average, 15.7% of Brachypodium and 11.3% barley kernels inoculated with microconidia developed symptoms. Full size image Similar results were obtained in infection assays with barley heads. On drop-inoculated barley heads, discolouration of glumes and other flowering tissues were observed on 11.1% of the kernels inoculated with microconidia ( Fig. 7b ). Under the same conditions, approximately 80% of barley kernels inoculated with macroconidia developed symptoms ( Fig. 7b ). Infection of unwounded barley heads by microconidia confirmed the infectivity of microconidia on floral tissues, although they are smaller and less efficient at plant infection than macroconidia. Microconidia are formed inside diseased rice plants Because microconidia are formed in submerged cultures, it is likely that they are also produced by M. oryzae inside diseased rice plants, particularly in the vascular system. To test this hypothesis, we first examined rice seedlings infected by wound inoculation with macroconidia of transformant GFP70. Healthy leaf sheath tissues adjacent to the diseased areas were collected from inoculated plants 7 d.p.i., washed and homogenized in sterile water by gentle grinding. After filtration through one layer of Miracloth followed by one layer of Whatman filter paper, the filtrates were centrifuged at 4,500 g . The resulting pellets were re-suspended in sterile water and examined by epifluorescence microscopy ( Fig. 8a ). Among the 21 samples examined, microconidia with GFP signals were readily observed in four of them ( Fig. 8a ). We repeated this experiment with barley heads drop-inoculated at the third kernel from the bottom. Microconidia with GFP signals were observed in the neck region below the diseased kernels sampled 14 days post inoculation ( Fig. 8a ). These data indicate that microconidia were produced inside rice and barley plants by the inoculating strain GFP70. In the other samples, no or only rare microconidium-like structures with GFP signals were observed. 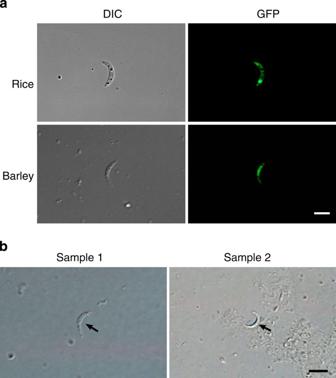Figure 8: Detection of microconidia produced in infected rice plants. (a) Rice leaf sheath and barley neck tissues adjacent to the diseased areas were collected from plants inoculated with GFP70 and examined under DIC (left) and epifluorescence (right) microscopy. GFP signals were observed in microconidia producedin planta. (b) Microconidia (arrows) were observed in tissues adjacent to the neck blast lesions in diseased rice plants collected from the fields in Liaoning province. Scale bar, 5 μm for (a,b). Figure 8: Detection of microconidia produced in infected rice plants. ( a ) Rice leaf sheath and barley neck tissues adjacent to the diseased areas were collected from plants inoculated with GFP70 and examined under DIC (left) and epifluorescence (right) microscopy. GFP signals were observed in microconidia produced in planta . ( b ) Microconidia (arrows) were observed in tissues adjacent to the neck blast lesions in diseased rice plants collected from the fields in Liaoning province. Scale bar, 5 μm for ( a , b ). Full size image To determine whether microconidia also are produced inside diseased rice plants in nature, plants with typical neck blast symptoms were collected from two fields in Liaoning province, China. Healthy stem tissues below the neck blast lesions and crown regions of each diseased rice plant were collected and homogenized in sterile water. After filtration through Miracloth and Whatman filter paper, the filtrates were concentrated by centrifugation before microscopic examination. Although the debris of ground plant tissues was problematic, microconidia or microconidium-like structures were observed in 8 of 28 samples examined ( Fig. 8b ). These results indicate that microconidia are produced by M. oryzae inside rice plants under the field conditions and they may be disseminated from the infected region to healthy parts without disease symptoms. Identification of genes uniquely expressed in microconidia To identify genes that were specifically or highly expressed in microconidia, we conducted RNA-Seq analysis with vegetative hyphae, macroconidia and microconidia of strain 70-15. To our surprise, transcripts representing over 5,000 M. oryzae genes were present in microconidia, which likely have limited metabolic activities. Most of these transcripts may be carried over from the phialides during microconidium formation. In comparison with macroconidia and vegetative hyphae, only seven genes (reads per kilobase of transcript per million-mapped reads >2) were found to be specifically expressed in microconidia and eight genes was increased over 20-folds in microconidia ( Supplementary Table 2 ). Two of them, encoding hypothetical proteins, were verified by PCR with reverse transcription (RT–PCR) to be specifically expressed in microconidia ( Supplementary Fig. 6 ) and may be suitable for the detection of microconidia in rice plants. Many filamentous ascomycetes produced macroconidia and microconidia that have different biological functions dependent on specific fungal species [20] . Although there is no experimental evidence, microconidia are hypothesized to function as spermatia during sexual reproduction in M. oryzae [6] , [7] . In this study, we showed that abundant microconidia were produced in submerged liquid cultures in the absence of the opposite mating type. The condition in submerged cultures does not support sexual reproduction and is more similar to in planta growth environment. In addition, germination of microconidia was independent of mating partners. Therefore, whether they function as spermatia or not, microconidia likely have other biological functions in M. oryzae , such as decimation and disease spreading. Interestingly, we found that microconidium production was inhibited in cultures that became heavily melanized due to nitrogen starvation after incubation at 25 °C for a week. Incubation as a lower temperature (20 °C) may stimulate microconidium production by reducing growth rate and avoiding the nitrogen starvation response. Germination of microconidia has not been previously observed in M. oryzae . Here we showed that approximately 5% and 10% of microconidia germinated on 1% water agar and plant leaves, respectively. The germination rate was consistently higher on leaf surfaces than on artificial surfaces in independent replicates, suggesting that certain plant surface chemicals may stimulate microconidium germination. In M. oryzae , germination of macroconidia is independent of surface signals but appressorium formation is triggered by the attachment to hydrophobic surfaces. In addition to physical signals recognized by germ tubes, plant surface chemicals, such as cutin monomers and primary alcohols, are known to induce appressorium formation [2] , [8] , [12] , [21] , [22] . It is possible that the difference between the germination rate on 1% water agar and leaf surface is related to certain physical and/or chemical signals of plant leaves. Although appressoria were not formed by microconidia, experimental approaches used to study plant surface signals recognized by macroconidia can be used in future studies to identify environmental cues recognized by microconidia. It will be important to determine whether cAMP or 3-isobutyl-1-methylxanthine treatment has any stimulatory effect on microconidium germination because surface recognition for appressorium formation by macroconidia is regulated by the cAMP–protein kinase A signalling pathway [8] , [12] . In M. oryzae , macroconidium germination is a very efficient process and germ tubes are formed in over 95% of macroconidia after incubation for 30 min. In contrast, germ tubes could be observed only in a small portion (<10%) of microconidia after incubation for 24 h or longer. In addition, we found that microconidium germination was more efficient on 1% water agar than on CM medium, indicating that nutrients had no stimulatory effects on microconidium germination. These differences between macroconidia and microconidia in the timing and conditions for germination may explain why microconidium germination was not observed in earlier studies [6] . Although in some fungi, such as Fusarium oxysporum and F. verticillioides , microconidia can germinate as efficiently as macroconidia, microconidium germination has not been observed in other fungal pathogens such as Botrytis cinerea and Sclerotinia sclerotiorum . Our results indicate that only a small portion of microconidia were able to germinate, probably due to the lack of mitochondria in most of them. In Neurospora crassa , microconidium germination is also observed only in some microconidia in cultures [20] . Interestingly, the majority of germinated microconidia failed to form colonies when they were transferred to nutrient medium. Microscopic examination revealed that many of the germinated microconidia became highly vacuolated and appeared to be dead by 120 h, and only approximately 20% of those that were still alive contained more than one nucleus. In M. oryzae, autophagy has been linked to the vacuolization and collapse of macroconidium compartments after appressorium formation [16] . However, cell death still occurred to germinated microconidia in the Mgatg1 mutant ( Supplementary Fig. 2 ), suggesting the involvement of other cell death mechanisms. In infection assays with intact rice or barley seedlings, microconidia failed to cause disease symptoms, which was consistent with our observation that appressoria were not formed by germ tubes from microconidia. In addition, with limited carbon storage in microconidia, there will not be enough energy reserve to generate sufficient turgor pressure even if appressoria are formed by microconidia. Therefore, it is not surprising that microconidia failed to infect intact plants. However, microconidia could infect and cause necrotic lesions on rice and other grass species through wounds under laboratory conditions. Under the field conditions, wounds caused by natural forces or insects may provide the infection sites for microconidia. Therefore, microconidia could be an important part of the rice blast disease cycle. It is well known that M. oryzae mutants defective in appressorium turgor generation or appressorial penetration can infect through wounds [2] , [8] . Germ tubes emerged from microconidia may use a similar strategy to invade plant cells via wounds. Nevertheless, it is possible that compounds produced by plants at the wounding sites may stimulate germination or virulence of microconidia in M. oryzae . On flowering Brachypodium and barley heads, the kernels inoculated with microconidia developed disease symptoms without intentional wounding other than gently pulling glumes open for drop inoculation. It is possible that floral tissues are more susceptible to microconidia due to the presence of virulence-stimulating compounds. For the wheat scab or head blight disease caused by F. graminearum , certain compounds in anthers are known to stimulate virulence of the pathogen and pre-dispose flowering heads to fungal infection [23] . The head blight disease symptom is similar between wheat scab and wheat blast. On rice plants, neck blast also occurs at the heading stage and blocks seed filling. Therefore, it is tempting to speculate that microconidia may be produced inside infected rice plants and dispersed to flowering heads. Specific compounds in floral tissues or certain environmental factors at the heading stage stimulate the virulence of microconidia and trigger the development of disease symptoms, which may be one of the reasons for the outbreaks of neck blast in the rice field without severe leaf blast symptoms (limited macroconidia). Therefore, it will be important to determine how M. oryzae microconidia invade and colonize floral tissues. Because macroconidia are not formed in submerged cultures, it is likely that only microconidia are produced by M. oryzae inside plant tissues. Diameter of smallest late metaxylem vessels in the leaf blade, leaf sheath and internode are 7, 13, 17 μm, respectively [24] . Due to their smaller size (0.7 μm in width on average) [7] , microconidia produced in planta may allow the pathogen to spread readily via the vascular system. As a hemibiotrophic pathogen, symptomless spreading of M. oryzae in rice plants has been reported [25] . Its ability to infect rice plants through roots also suggested the possibility of systemic infection by this pathogen [26] . However, these studies could not rule out macroconidium contamination from diseased areas [27] . In this study, we were able to detect microconidia in the healthy parts of rice plants with leaf or neck blast symptoms that were artificially inoculated in the greenhouse or collected from rice fields, suggesting that microconidia may play a role in the disease cycle of M. oryzae . However, to determine the importance of microconidia in the epidemiology of rice blast, it will be important and necessary to conduct root infection assays with mutants that are blocked in the production of macroconidia but still form microconidia. For wheat blast, the primary inoculum for head infection is unknown [28] , and it will be important to determine whether microconidia are present in the neck, rachis or other head tissues of plants with wheat blast symptoms. Severe wheat blast outbreaks without blast symptoms on leaves may be related to tissue-specific symptoms caused by microconidia transported to wheat heads. Therefore, results from this study are important to better understand and control rice blast, wheat blast and other diseases caused by Magnaporthe species. Strains and culture conditions The wild type and mutant strains of Magnaporthe oryzae used in this study ( Supplementary Table 3 ) were cultured on oatmeal agar plates at 25 °C under fluorescent light for the production of macroconidia as described [15] , [21] . Strain GFP70 expressing GFP in the cytoplasm was generated by transforming pRM7 (ref. 29 ) containing the P RP27 -GFP construct into 70-15. Expression of GFP had no effect on growth, differentiation and plant infection. For infection assays, macroconidia were harvested from 10-day-old cultures and re-suspended to 5 × 10 5 ml −1 in 0.25% gelation. Production of microconidia on oatmeal agar cultures was assayed as described [6] . For production of microconidia in liquid cultures, two blocks of 10-day-old oatmeal cultures were cut out with a 5-mm diameter core borer and used to inoculate 40 ml of home-made PDB, CM and 5 × yeast extract–glucose (YEG) [21] . After incubation at 25 °C or 20 °C for 4–7 days, microconidia were harvested by filtration through two layers of Miracloth (CalBiochem) and followed by filtration through one layer of Whatman filter paper (medium, GE Healthcare). Assays for germination and appressorium formation Freshly harvested microconidia were washed once by centrifugation at 4,500 g for 10 min and re-suspended in sterile distilled water to the final concentration of 10 7 microconidia per ml. After spreading 1 ml of microconidium suspensions on each plates of 1% water agar, CM and 5 × YEG, microconidium germination was examined after incubation at 20, 25 or 30 °C for 1, 2 and 3 days. For assaying microconidium germination on plant surfaces, the second leaves of 8-day-old barley seedlings were inoculated with microconidium suspensions by drop-inoculation as described [21] . Microconidium germination and appressorium formation were examined with a Olympus BX-53 microscope after peeling off barley epidermal layers as described [14] . Plant infection assays Microconidia harvested from PDB cultures were re-suspended to 1 × 10 7 ml −1 in 0.25% gelation and used for spray and injection infection assays with 2-week-old seedlings of rice cultivars Nipponbare or Lijiangxintuanheigu and 10-day-old seedlings of barley cultivar Golden Promise [14] , [30] . Lesion formation was examined 7 days post inoculation. For abrasion and cutting infection assays, rice or barley leaves were abraded with an emery board or scratched with a needle before being inoculated with small drops (20 μl) of spore suspensions [14] . Inoculated plants were placed in a dew chamber for 48 h and then transferred to the growth chamber with a photoperiod of 16 h. Lesions were examined 10 d.p.i. For infection assays with Brachypodium (BD-21) and barley (Golden Promise) heads, suspensions of macroconidia (5 × 10 5 ml −1 ) and microconidia (10 7 ml −1 ) were pipetted into randomly selected kernels after gently pulling the glumes apart. Inoculated heads were then covered with a small plastic bag, which was removed after 2 days. Disease symptoms were examined after growing in a growth chamber for another 7–14 days. Nucleus and mitochondrion staining For nucleus staining, freshly harvested microconidia were re-suspended to 5 × 10 6 ml −1 in 0.1 M phosphate-buffered saline buffer (pH 6.8). After staining with 20 μg ml −1 of 4′,6-diamidino-2-phenylindole (Sigma) for 7 min, microconidia were washed twice with 0.1 M phosphate-buffered saline buffer before microscopic examination. Mitochondria were stained with the MitoTracker Red FM (Invitrogen) following the instruction provided by the manufacturer. After staining for 30 min at 28 °C, microconidia were washed five times with sterile water and examined under an Olympus BX-53 microscope. Microconidia germinated on 1% water agar were stained with the Hoechst Stain Kit (Beyotime, Shanghai, China). Lipid body and glycogen staining Freshly harvested macroconidia and microconidia were stained with Nile Red (Sigma-Aldrich, St Louis) to visualize lipid bodies as described [31] . Stained samples were washed once with distilled water by centrifugation before microscopical examination. Glycogens were stained with a solution prepared by dissolving 60 mg of KI and 10 mg of I 2 in 1 ml of distilled water as described [31] , [32] . Electron microscopy examination Samples for SEM or TEM were fixed in 4% (v/v) glutaraldehyde in 0.1 M phosphate buffer (pH 6.8) for 12 h at 4 °C and dehydrated in a series of acetone (30, 50, 70, 80, 90 and 100%; vol/vol). For assaying microconidium germination on plant surface, barley leaves were mounted on stubs and sputter-coated with gold–palladium before examination with a Hitachi S-4800 SEM microscope at 5 kV (Jeol, Tokyo). For TEM examination, microconidium samples were infiltrated and embedded with LR White Resin (Sigma-Aldrich, St Louis, MO, USA). Ultra-thin sections were prepared and treated with uranyl acetate and lead citrate before examination with a Hitachi HT7700 TEM at 80 KV as described [32] . RNA-Seq analysis and RT–PCR verification For RNA isolation, vegetative hyphae were harvested from 2-day-old 5 × YEG cultures as described [21] . Microconidia from 7-day-old PDB cultures and macroconidia from 10-day-old oatmeal plates were prepared as described above. Total RNA was isolated with the Qiagen RNeasy Plant Mini kit. Library construction with the TruSeq RNA Sample Preparation Kit (Illumina) and sequencing with an Illumina HiSeq 2000 sequencer were performed at BGI-Shenzhen. For each sample, at least 7 Mb high-quality reads were obtained. The cleared reads were mapped to the corresponding M. oryzae 70-15 genes with the Short Oligonucleotide Analysis Package (SOAP) v2.21 program ( http://soap.genomics.org.cn ). Transcript abundances were normalized based on the expected reads per kilobase of exon per million fragments mapped (RPKM). Genes with false discovery rate ≤0.001 and fold change ≥2 were identified as differentially expressed genes as described [33] . For RT–PCR analysis, primers 5′-CTTCTCATTCGTCCTC-3′ and 5′-CCACAGGTCGTAGTCT-3′ were used for MGG_09130, and primers 5′-TGCGTTCCGTGTGAGAGT-3′ and 5′-ACATCCGAGCACACCATC-3′ for MGG_02339. Accession codes : The RNA-Seq data have been deposited in the NCBI Sequence Read Archive database with accession code SRP044698 . How to cite this article: Zhang, H. et al. Germination and infectivity of microconidia in the rice blast fungus Magnaporthe oryzae . Nat. Commun. 5:4518 doi: 10.1038/ncomms5518 (2014).